RNase ZS1processesUbL40mRNAs and controls thermosensitive genic male sterility in rice Thermosensitive genic male-sterile (TGMS) lines, which are male-sterile at restrictive (high) temperatures but male-fertile at permissive (low) temperatures, have been widely used in breeding two-line hybrid rice ( Oryza sativa L.). Here we find that mutation of thermosensitive genic male sterile 5 ( tms5 ) in rice causes the TGMS trait through a loss of RNase Z S1 function. We show that RNase Z S1 processes the mRNAs of three ubiquitin fusion ribosomal protein L40 ( Ub L40 ) genes into multiple fragments in vitro and in vivo . In tms5 mutants, high temperature results in increased levels of Ub L40 mRNAs. Overaccumulation of Ub L40 mRNAs causes defective pollen production and male sterility. Our results uncover a novel mechanism of RNase Z S1 -mediated Ub L40 mRNA regulation and shows that loss of this regulation produces TGMS in rice, a finding with potential applications in hybrid crop breeding. Hybrid rice, which yields ~10–20% more grain than conventional rice, has been planted in ~60% (~17 million hectares) of the rice-growing area in China and is also cultivated in many other countries, thus providing a key component of the global food supply [1] , [2] , [3] . Rice is strictly self-pollinating; therefore, hybrid varieties are bred using male-sterile maternal lines that fail to produce viable pollen, thus preventing self-pollination. Hybrid rice breeding uses the well-developed three-line and two-line systems [4] , [5] . The three-line system uses a cytoplasmic male-sterile (CMS) line, a restorer line and a CMS maintainer line to produce F 1 hybrid seeds and maintain the CMS line [6] , [7] , [8] . Three-line hybrid rice has been grown since the 1970s and is a major type of hybrid rice [1] , [4] , [9] . However, the limited germplasm resources of restorer lines and the genetic diversity between CMS and restorer lines have limited further improvements in three-line breeding [10] . The two-line breeding system uses thermosensitive genic male sterility (TGMS) lines or photoperiod-sensitive genic male sterility (PGMS) lines as maternal parents to produce hybrid seeds. TGMS and PGMS lines are male-sterile under restrictive conditions (high temperatures for TGMS and long-day for PGMS) but convert to male-fertile under permissive conditions (low temperatures for TGMS and short-day for PGMS); thus, they can self-pollinate under permissive conditions [10] , [11] . The TGMS and PGMS traits are controlled by nuclear, recessive genes and most normal rice cultivars can restore male fertility, thus providing broader genetic resources for rice breeding to produce hybrids with strong hybrid vigour [10] , [11] , [12] . Two-line hybrid rice has been planted in China since 1993 and over 3.4 million hectares were grown in 2011 ( Supplementary Fig. 1 ). AnnongS-1 (AnS-1), the first indica rice ( Oryza. sativa ssp. indica ) TGMS line, was found in 1987 as a spontaneous mutant [13] . AnS-1 and its derived TGMS lines have been widely used for two-line hybrid rice breeding, and their TGMS trait is controlled by a single recessive locus, tms5 (ref. 13 ). A candidate region on the short arm of chromosome 2 has been reported [14] , [15] , [16] , [17] ; however, the identity of the TMS5 gene has not been confirmed and the molecular mechanism by which it produces male sterility remains unclear. Here we report that tms5 confers the TGMS trait through a loss-of-function mutation in the gene coding for RNase Z S1 , which regulates Ub L40 mRNA levels during male development. Our results uncover a novel mechanism of RNase Z S1 -mediated Ub L40 mRNA processing, which controls TGMS in rice and has potential applications in hybrid crop breeding. AnS-1 and Zhu1S are temperature-sensitive TGMS lines Zhu1S is one of the indica TGMS lines frequently used for commercial two-line hybrid rice breeding ( Supplementary Fig. 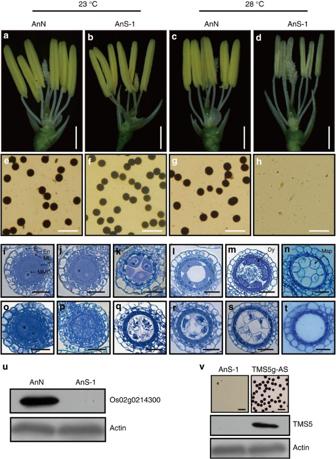Figure 1: Phenotypes and complementation of AnS-1. (a–h) Anther morphology and pollen fertility of AnN and AnS-1. Normal anthers (a,b) and pollen (e,f) in AnN and AnS-1 at the permissive temperature (23 °C). Normal anthers (c) and pollen (g) in AnN and abnormal anthers (d) and abortive pollen (h) in AnS-1 grown at the restrictive temperature (28 °C). (i–t) Comparison of transverse sections of anthers of AnS-1 grown at 23 °C (i–n) and 28 °C (o–t). At 23 °C, the MMCs underwent meiosis to produce microspores (immature pollen grains); at 28 °C, few or no microspores were generated. (i,o) Early MMC stage; (j,p) late MMC stage; (k,q) meiotic leptotene stage; (l,r) meiotic pachytene stage; (m,s) dyad stage; (n,t) young microspore stage. E, epidermis; En, endothecium; ML, middle layer; T, tapetum; MMC, microspore mother cell, Dy, dyad; Msp, microspore. Scale bars, 1 mm (a–d), 100 μm (e–h) and 20 μm (i–t). (u) The protein encoded by Os02g0214300 could not be detected in AnS-1 by immunoblot analysis. The constitutively expressed rice Actin protein was used as an internal control. (v) Pollen fertility was restored in the AnS-1 background containingTMS5genomic DNA (TMS5g-AS) grown at the restrictive temperature (28 °C; above, right). No pollen was produced in anthers of AnS-1 grown under the same conditions (above, left). TMS5 protein was detected in TMS5g-AS line but not in AnS-1 (middle). The Actin protein was used as an internal control. 1 and Supplementary Table 1 ). 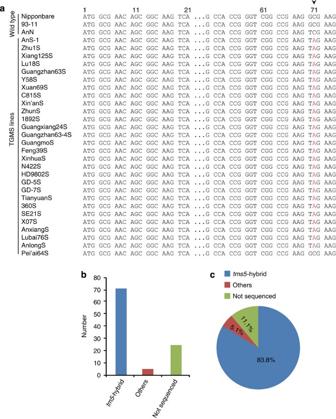Figure 2: Application oftms5in two-line hybrid rice breeding. (a) Left, names of wild-type and TGMS lines. Right, alignment of 75 base-pair DNA sequence of the coding region ofTMS5in wild-type and different TGMS lines. Nucleotide numbers within theTMS5-coding sequence are shown at the top. The mutated nucleotide at position 71 (arrowed) intms5lines is shown in red. (b) Number of different two-line hybrid rice cultivars bred using tms5-TGMS lines (tms5-hybrid) compared with other two-line hybrid rice cultivars grown in China in 2011 (left figure). Proportions of the two-line hybrid rice-growing area (B3.4 million hectares) planted with tms5-hybrid cultivars and other hybrid cultivars bred with others and non-sequenced T/PGMS lines in China in 2011 (right figure). (c) Proportions of the two-line hybrid rice-growing area (~3.4 million hectares) planted withtms5-hybrid cultivars and other hybrid cultivars bred with others and non-sequenced T/PGMS lines in China in 2011. To examine the phenotype of AnS-1 and Zhu1S in detail, growth chambers and Phytotrons were used to grow plants under fixed photoperiod conditions and at different day average temperatures (DAT; See Methods and Supplementary Table 2a,b ). AnS-1 and Zhu1S were grown in the field until the panicle length was ~1 cm and then the plants were transferred into growth chambers or Phytotrons for 2–3 weeks, respectively. At the permissive temperature (~23 °C DAT), AnS-1 is male-fertile, similar to the normal male-fertile line AnnongN (AnN, a parental line of AnS-1). At restrictive temperatures, AnS-1 becomes male-sterile, producing abortive pollen grains at ~26 °C DAT, and no pollen grains at 28 °C or higher DAT ( Fig. 1a–h and Supplementary Fig. 2a ). At 23 °C, AnS-1 developed normally ( Fig. 1i–n ), whereas at 28 °C few microspore mother cells (MMCs) undergo normal meiosis, and any microspores that are produced eventually disintegrate ( Fig. 1o–t ). By contrast, the day length had little effect on male sterility of AnS-1 ( Supplementary Fig. 2 ). We observed a similar phenotype in Zhu1S grown at the restrictive temperatures of >23 °C DAT ( Supplementary Fig. 3 ). Figure 1: Phenotypes and complementation of AnS-1. ( a – h ) Anther morphology and pollen fertility of AnN and AnS-1. Normal anthers ( a , b ) and pollen ( e , f ) in AnN and AnS-1 at the permissive temperature (23 °C). Normal anthers ( c ) and pollen ( g ) in AnN and abnormal anthers ( d ) and abortive pollen ( h ) in AnS-1 grown at the restrictive temperature (28 °C). ( i – t ) Comparison of transverse sections of anthers of AnS-1 grown at 23 °C ( i – n ) and 28 °C ( o – t ). At 23 °C, the MMCs underwent meiosis to produce microspores (immature pollen grains); at 28 °C, few or no microspores were generated. ( i , o ) Early MMC stage; ( j , p ) late MMC stage; ( k , q ) meiotic leptotene stage; ( l , r ) meiotic pachytene stage; ( m , s ) dyad stage; ( n , t ) young microspore stage. E, epidermis; En, endothecium; ML, middle layer; T, tapetum; MMC, microspore mother cell, Dy, dyad; Msp, microspore. Scale bars, 1 mm ( a – d ), 100 μm ( e – h ) and 20 μm ( i – t ). ( u ) The protein encoded by Os02g0214300 could not be detected in AnS-1 by immunoblot analysis. The constitutively expressed rice Actin protein was used as an internal control. ( v ) Pollen fertility was restored in the AnS-1 background containing TMS5 genomic DNA (TMS5g-AS) grown at the restrictive temperature (28 °C; above, right). No pollen was produced in anthers of AnS-1 grown under the same conditions (above, left). TMS5 protein was detected in TMS5g-AS line but not in AnS-1 (middle). The Actin protein was used as an internal control. Full size image Cloning the gene associated with TGMS in AnS-1 and Zhu1S To clone tms5 and the gene conferring the TGMS trait in Zhu1S, we developed and characterized two mapping populations (see Methods, Supplementary Fig. 4a,c ), both of which narrowed the target locus to the same region on the short arm of chromosome 2 ( Supplementary Fig. 4a,d ). Sequencing of the mapped region in the male-sterile lines AnS-1 and Zhu1S revealed a C-to-A transition at position 71 of the gene Os02g0214300 compared with that in AnN, creating a premature stop codon ( Supplementary Fig. 4b,e ). This change is identical to the premature stop codon mutation mapped to the same gene in the ptgms2-1 locus [18] . The protein encoded by Os02g0214300 was detected by immunoblotting in AnN, but not in AnS-1 ( Fig. 1u ). Therefore, we considered Os02g0214300 to be a candidate gene for TMS5. For genetic complementation to verify that Os02g0214300 indeed corresponds to TMS5 , genomic DNA fragments harbouring Os02g0214300 from AnN and the rice cultivar Nipponbare ( O. sativa ssp. japonica ) were transformed into the tms5 AnS-1 and Zhu1S lines, respectively. Male fertility was restored in transgenic plants of AnS-1 (designated TMS5g-AS) and Zhu1S (designated TMS5g-ZS) at the restrictive temperature ( Fig. 1v , Supplementary Fig. 5 ). Moreover, knockdown of TMS5 by RNA interference (RNAi) in the japonica lines Zhonghua11 (ZH11; designated TMS5i-ZH, Supplementary Fig. 6a–d ) and Nipponbare (designated TMS5i-NB, Supplementary Fig. 6e–f ) showed similar pollen abortion as in AnS-1 and Zhu1S at restrictive temperatures. These results demonstrate that the loss-of-function mutation of TMS5 confers the TGMS phenotype in AnS-1 and Zhu1S. tms5 is a major TGMS gene widely used in rice breeding Dozens of TGMS lines are used in two-line hybrid rice breeding [19] . To explore whether other TGMS lines also harbour a tms5 mutation, we sequenced the TMS5 locus in 25 other widely used TGMS lines and found that 24 of them carried the same tms5 mutation ( Fig. 2a ). In 2011, 71 commercial two-line hybrid rice cultivars bred with tms5 -containing TGMS lines accounted for at least 71% of all two-line hybrid rice cultivars and 83.8% (~2.9 million hectares) of all the land used to grow two-line hybrid rice in China ( Fig. 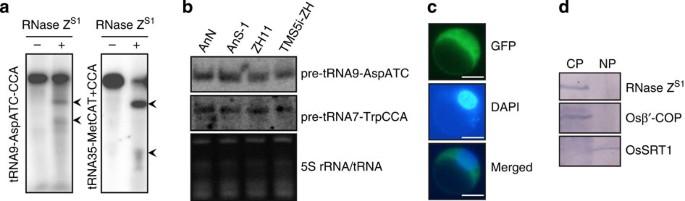Figure 3: RNase ZS1processes tRNA invitroand localizes in the cytoplasm. (a) Recombinant His-tagged RNase ZS1processed the 3′ ends of both tRNA9-AspATC-CCA and tRNA35-MetCAT+CCAin vitro. Arrows indicate the processed product bands. (b) RNA blot analysis showed no obvious difference in tRNA precursor accumulation in wild-type (AnN and ZH11), AnS-1 and TMS5i-ZH plants. 5S rRNA/tRNA stained with ethidium bromide was used as a loading control. (c) RNase ZS1-GFP (green) was observed in the cytoplasm (top) but not in the nucleus (middle, stained with DAPI, blue). Scale bars, 10 μm. (d) RNase ZS1was detected in cytoplasmic protein extracts using immunoblot analysis. Osβ′-COP and OsSRT1 were used as the indicators of cytoplasmic and nuclear protein controls, respectively. CP, cytoplasmic proteins; NP, nuclear proteins. 2b,c and Supplementary Table 3 ). Accordingly, tms5 serves as the major TGMS genetic resource for two-line hybrid rice breeding. Figure 2: Application of tms5 in two-line hybrid rice breeding. ( a ) Left, names of wild-type and TGMS lines. Right, alignment of 75 base-pair DNA sequence of the coding region of TMS5 in wild-type and different TGMS lines. Nucleotide numbers within the TMS5 -coding sequence are shown at the top. The mutated nucleotide at position 71 (arrowed) in tms5 lines is shown in red. ( b ) Number of different two-line hybrid rice cultivars bred using tms5-TGMS lines ( tms5 -hybrid) compared with other two-line hybrid rice cultivars grown in China in 2011 (left figure). Proportions of the two-line hybrid rice-growing area (B3.4 million hectares) planted with tms5-hybrid cultivars and other hybrid cultivars bred with others and non-sequenced T/PGMS lines in China in 2011 (right figure). ( c ) Proportions of the two-line hybrid rice-growing area (~3.4 million hectares) planted with tms5 -hybrid cultivars and other hybrid cultivars bred with others and non-sequenced T/PGMS lines in China in 2011. Full size image TMS5 encodes a conserved RNase Z protein TMS5 encodes an evolutionarily conserved ribonuclease Z (RNase Z), which occurs in almost all kingdoms of life [20] , [21] , [22] . Two forms of RNase Z exist in eukaryotes, the short form (RNase Z S ) and the long form (RNase Z L ; Supplementary Fig. 7 ), while prokaryotes only have RNase Z S (refs 20 , 22 ). The TMS5 protein, with 302 amino acids, belongs to the short-form group and we refer to it as RNase Z S1 . In rice, RNase Z S1 is constitutively expressed in various tissues ( Supplementary Fig. 8a ). At the protein level, RNase Z S1 accumulated stably at both permissive and restrictive temperatures ( Supplementary Fig. 8b ). In anther, its mRNA expression was relatively enriched in MMCs and this did not change at low (23 °C) and high (28 °C) temperatures ( Supplementary Fig. 8c,d ). These results indicate that RNase Z S1 itself is temperature-insensitive. RNase Z S1 is cytoplasmic and processes tRNAs in vitro RNase Z proteins process the 3′ ends of tRNAs [21] , [23] , [24] , [25] . The CCA sequence in 3′ terminal of the tRNA is critical for tRNA maturation and function. RNase Z mainly processes CCA-less pre-tRNAs; however, it can process CCA-containing pre-tRNAs in the nucleus or mitochondria [26] , [27] . To investigate the enzymatic activity of RNase Z S1 , we tested whether RNase Z S1 cleaved two pre-tRNAs, pre-tRNA9-AspATC (without CCA) and pre-tRNA35-MetCAT (with CCA). We expressed recombinant RNase Z S1 in Escherichia coli ( E. coli ) and found that it processed the 3′ ends of both pre-tRNAs, with or without CCA, in vitro ( Fig. 3a ), indicating that RNase Z S1 possesses endonuclease activity. We then examined the in vivo accumulation of mature and precursor tRNA in AnN, AnS-1, ZH11 and TMS5i-ZH but found no obvious difference between wild-type and tms5 plants ( Fig. 3b and Supplementary Fig. 9a ). The mature tRNA levels were unchanged at permissive or restrictive temperatures when analysed in NIL5 and NIL8 (near-isogenic lines 5 and 8 of Zhu1S in the background of the indica cultivar 93-11) and 93-11 ( Supplementary Fig. 9b ). These results indicate that RNase Z S1 does not affect tRNA 3′ end processing in vivo . Figure 3: RNase Z S1 processes tRNA in vitro and localizes in the cytoplasm. ( a ) Recombinant His-tagged RNase Z S1 processed the 3′ ends of both tRNA9-AspATC-CCA and tRNA35-MetCAT+CCA in vitro . Arrows indicate the processed product bands. ( b ) RNA blot analysis showed no obvious difference in tRNA precursor accumulation in wild-type (AnN and ZH11), AnS-1 and TMS5i-ZH plants. 5S rRNA/tRNA stained with ethidium bromide was used as a loading control. ( c ) RNase Z S1 -GFP (green) was observed in the cytoplasm (top) but not in the nucleus (middle, stained with DAPI, blue). Scale bars, 10 μm. ( d ) RNase Z S1 was detected in cytoplasmic protein extracts using immunoblot analysis. Osβ′-COP and OsSRT1 were used as the indicators of cytoplasmic and nuclear protein controls, respectively. CP, cytoplasmic proteins; NP, nuclear proteins. Full size image To explore where RNase Z S1 localizes, we expressed RNase Z S1 -GFP (green fluorescent protein) in rice protoplasts and found that it localizes in the cytoplasm but not in the nucleus ( Fig. 3c ). This observation was further verified by immunoblot analysis of partially purified nuclear and cytoplasmic proteins ( Fig. 3d ). Therefore, we propose that RNase Z S1 functions in the cytoplasm but does not act in tRNA processing in the nucleus. Ub L40 mRNAs accumulate in tms5 plants at high temperature To further address whether RNase Z S1 has a role in mRNA metabolism in the cytoplasm, we performed independent whole-genome microarray and RNA-seq analyses, using RNA from young panicles (flower inflorescences) of wild-type lines (AnN, ZH11 and 93-11) and tms5 or RNase Z S1 knockdown lines (AnS-1, TMS5i-ZH, NIL5 and NIL8) grown at permissive and restrictive temperatures. These analyses identified three common mRNAs that accumulate at higher levels in tms5 plants at the restrictive but not the permissive temperature ( Fig. 4a,b ; Supplementary Fig. 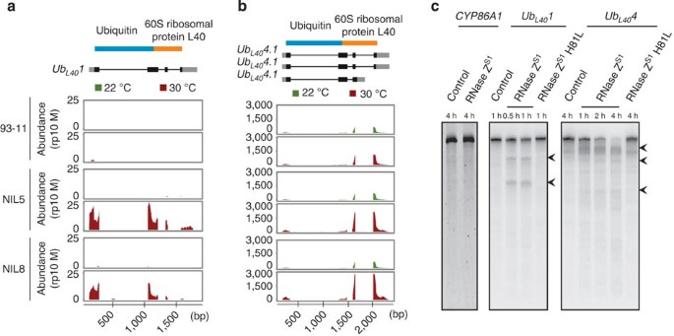Figure 4:UbL401andUbL404mRNAs accumulate intms5plants at high temperature. (a,b) Overaccumulation ofUbL401andUbL404mRNAs intms5plants at the restrictive temperature. RNA-seq profile ofUbL401(a) andUbL404(b) in 93-11, NIL5 and NIL8 (near-isogenic line 5 and line 8 of Zhu1S-derivedtms5in 93-11 background) at 22 and 30 °C. The ubiquitin domain and 60S ribosomal protein L40 domain are shown as blue and orange boxes, respectively. Transcripts ofUbL401(one mRNA isoform) andUbL404(three mRNA isoforms) are shown with thick boxes representing exons, thin lines representing introns and grey boxes representing untranslated regions (UTRs). Wiggle plots of RNA-seq data represent reads per 10 million (rp10M). (c)In vitroprocessing ofCYP86A1(left, a negative control),UbL401(middle) andUbL404(right) mRNAs by recombinant wild-type RNase ZS1and enzymatic null (RNase ZS1H81L), respectively. The assay time is marked above the lanes. Arrows indicate bands processed by RNase ZS1. 10a and Supplementary Table 4 ). These mRNAs are from genes of the conserved ubiquitin-60S ribosomal protein L40 family ( Ub L40 ), namely Ub L40 1 ( Os09g0452700 ), Ub L40 2 ( Os03g0259500 ) and Ub L40 4 ( Os09g0483400 ; Supplementary Fig. 11 ). At the permissive temperature, Ub L40 1 , Ub L40 2 and Ub L40 4 mRNA levels were similar in wild-type and tms5 plants; at the restrictive temperature, the expression of these three genes, especially Ub L40 1 , was dramatically elevated in tms5 but not in wild-type plants ( Fig. 4a,b ; Supplementary Figs 10a, 12a and 13 ). Furthermore, Ub L40 1 , Ub L40 2 and Ub L40 4 preferentially expressed in stamens and were largely induced by restrictive temperature in tms5 stamens but not in other tissues ( Supplementary Fig. 12b–e ). Thus, accumulation of Ub L40 1 , Ub L40 2 and Ub L40 4 transcripts is temperature-sensitive in the tms5 background, and RNase Z S1 -dependent, suggesting that RNase Z S1 might be involved in processing Ub L40 mRNAs. Figure 4: Ub L40 1 and Ub L40 4 mRNAs accumulate in tms5 plants at high temperature. ( a , b ) Overaccumulation of Ub L40 1 and Ub L40 4 mRNAs in tms5 plants at the restrictive temperature. RNA-seq profile of Ub L40 1 ( a ) and Ub L40 4 ( b ) in 93-11, NIL5 and NIL8 (near-isogenic line 5 and line 8 of Zhu1S-derived tms5 in 93-11 background) at 22 and 30 °C. The ubiquitin domain and 60S ribosomal protein L40 domain are shown as blue and orange boxes, respectively. Transcripts of Ub L40 1 (one mRNA isoform) and Ub L40 4 (three mRNA isoforms) are shown with thick boxes representing exons, thin lines representing introns and grey boxes representing untranslated regions (UTRs). Wiggle plots of RNA-seq data represent reads per 10 million (rp10M). ( c ) In vitro processing of CYP86A1 (left, a negative control), Ub L40 1 (middle) and Ub L40 4 (right) mRNAs by recombinant wild-type RNase Z S1 and enzymatic null (RNase Z S1 H81L), respectively. The assay time is marked above the lanes. Arrows indicate bands processed by RNase Z S1 . Full size image RNase Z S1 processes mRNAs of Ub L40 genes To address this hypothesis, we transcribed Ub L40 1 , Ub L40 2 and Ub L40 4 RNAs in vitro and incubated the RNAs with recombinant RNase Z S1 proteins. All three Ub L40 mRNAs were processed into multiple fragments by the wild-type but not the enzymatic null RNase Z S1 proteins in vitro ( Fig. 4c , Supplementary Fig. 10b ). Furthermore, we employed RNA ligase-mediated 5′ rapid amplification of cDNA ends (RNA ligase-mediated-5′RACE) and mapped multiple degradation sites in the Ub L40 1 mRNA of wild-type plants (ZH11, AnN and 93-11) but not in AnS-1 and NIL5 ( Supplementary Fig. 14 ), suggesting that RNase Z S1 is involved in the processing of Ub L40 1 mRNA in vivo . We hypothesize that RNase Z S1 may recognize the secondary or tertiary structure of the target mRNAs and process them. Thus, we propose that at restrictive temperatures, the loss-of-function mutation of RNase Z S1 in tms5 plants results in unprocessed Ub L40 1 , Ub L40 2 and Ub L40 4 RNAs and the excess Ub L40 transcripts might lead to abnormal male development in the anther. Ub L40 genes are expressed in MMCs To further test our hypothesis, we examined the spatial and temporal expression of Ub L40 genes by in situ mRNA hybridization. In wild-type anthers, compared with sense probe signals, antisense probes of Ub L40 1 and Ub L40 4 detected stronger signals in MMCs than in other cell layers ( Fig. 5a,b ). In addition, Ub L40 1 , Ub L40 2 and Ub L40 4 expression levels were similar between high (28 °C DAT) and low (23 °C DAT) temperatures in wild type ( Fig. 5c and Supplementary Fig. 15 ). In contrast, all three Ub L40 genes tested showed stronger signals in MMCs at high temperature than in the RNase Z S1 mutants at low temperature, indicating the interplay between RNase Z S1 and Ub L40 mRNAs in male fertility ( Fig. 5d and Supplementary Fig. 15 ). Among the Ub L40 family members, Ub L40 4 may have a major role in the regulation of thermosensitive genic male sterility since the expression level of Ub L40 4 was much higher than that of Ub L40 1 and Ub L40 2 , consistent with the RNA-seq data in NIL5 and NIL8, and RT–PCR data in AnS-1 ( Figs 4a,b and 5d ; Supplementary Figs 10, 12, 13 and 15 ). 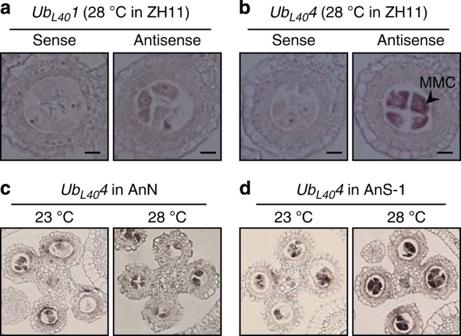Figure 5:UbL401andUbL404mRNAs preferentially express in MMCs. (a,b)In situhybridization ofUbL401(a) andUbL404(b) transcripts in anther. (c,d) At indicated temperatures, expression level ofUbL404in MMCs under high (28 °C) and low (23 °C) temperature in AnN (c) and AnS-1 (d). Scale bars, 10 μm (a,b). MMC, microspore mother cells. Figure 5: Ub L40 1 and Ub L40 4 mRNAs preferentially express in MMCs. ( a , b ) In situ hybridization of Ub L40 1 ( a ) and Ub L40 4 ( b ) transcripts in anther. ( c , d ) At indicated temperatures, expression level of Ub L40 4 in MMCs under high (28 °C) and low (23 °C) temperature in AnN ( c ) and AnS-1 ( d ). Scale bars, 10 μm ( a , b ). MMC, microspore mother cells. Full size image Overexpression of Ub L40 1 and 4 leads to male sterility To test whether the accumulation of Ub L40 1 and Ub L40 4 in tms5 plants could affect male fertility, we generated Ub L40 1 - and Ub L40 4 -overexpressing transgenic plants in the ZH11 background (designated Ub L40 1OE and Ub L40 4OE). These plants produced higher levels of Ub L40 1 and Ub L40 4 mRNAs than ZH11 and exhibited partial pollen abortion ( Supplementary Fig. 16 ), mimicking the phenotypes of tms5 lines at restrictive temperatures. Furthermore, we created Ub L40 1 or Ub L40 4 knockdown plants in the tms5 background, designated Ub L40 1i and Ub L40 4i. At restrictive temperatures, these plants exhibited reduced levels of Ub L40 1 and Ub L40 4 mRNAs and partially restored male fertility ( Supplementary Fig. 17 ). Thus, we hypothesize that regulation of Ub L40 mRNA levels by RNase Z S1 is critical for MMC development at high temperature in rice. Male sterility has been extensively applied to the breeding of crops for hybrid vigour, and these hybrids have larger stature and higher yields than the parent inbred lines. In rice, CMS lines and TGMS/PGMS lines are widely used in three-line and two-line hybrid rice breeding, respectively. Here we uncovered the molecular mechanism of rice TMS5, which functions in RNase Z S1 -mediated Ub L40 mRNA regulation during male development ( Fig. 6 ). At the permissive temperature, the level of Ub L40 mRNAs remains low in the tms5 mutant plants, allowing the production of normal pollen. At restrictive temperature, however, Ub L40 mRNAs are not processed by RNase Z S1 and their high level cause male sterility. The preferential expression of Ub L40 1, Ub L40 2 and Ub L40 4 in MMCs indicates that these mRNAs are crucial for MMC development. We notice that overexpression of Ub L40 1 and Ub L40 4 in wild type leads to male sterility without causing any other obvious defects. We hypothesize that additional factors that are restricted to the MMC might be required to assist Ub L40 genes in their functions ( Fig. 6 ). Our results thus uncover a novel function for the RNase Z S1 family, deepening our understanding of the molecular genetic basis of TGMS in rice. These findings have profound implications for hybrid breeding in crops. 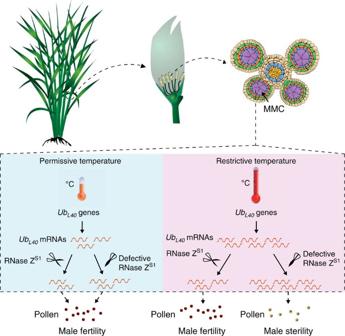Figure 6: A functional model for RNase ZS1controlling TGMS in rice. In rice anther,UbL40genes preferentially express in MMCs (in purple).UbL40mRNAs are induced by high (restrictive) temperature. In wild type, RNase ZS1processes mRNAs ofUbL40and maintains them at normal levels. In RNase ZS1defective mutant plants, excessive mRNAs ofUbL40accumulate in anthers and lead to male sterility. MMC, microspore mother cells. Figure 6: A functional model for RNase Z S1 controlling TGMS in rice. In rice anther, Ub L40 genes preferentially express in MMCs (in purple). Ub L40 mRNAs are induced by high (restrictive) temperature. In wild type, RNase Z S1 processes mRNAs of Ub L40 and maintains them at normal levels. In RNase Z S1 defective mutant plants, excessive mRNAs of Ub L40 accumulate in anthers and lead to male sterility. MMC, microspore mother cells. Full size image Male reproduction is very sensitive to alterations in environmental conditions. A long non-coding RNA (lncRNA), the long-day-specific male-fertility-associated RNA, causes a PGMS trait and was identified in Nongken58S [11] . At the same locus in the indica line Pei’ai64S, a non-coding RNA producing small RNAs was shown to confer a P/TGMS trait [10] . In addition, a temperature-sensitive splicing defect of the transcript encoding UDPase leads to male sterility in rice at high temperature [28] , [29] . Our results show that, in tms5 mutants, high temperature induces accumulation of Ub L40 mRNAs in MMCs and causes male sterility. It is possible that environmental conditions such as temperature and photoperiod may affect RNA metabolism at the post-transcriptional level. Defects in these processes might be harmful to the cells in anther development, leading to male sterility. The endonuclease RNase Z exhibits two forms, RNase Z S and RNase Z L , which are evolutionarily conserved in almost all organisms [21] , [22] . RNase Z proteins have various RNA substrates, including tRNAs and mRNAs. Different RNase Z proteins might process different substrates and functions in different subcellular compartments [21] . In prokaryotes, RNase Z S is involved in tRNA 3′ terminal processing and has a role in mRNA decay [30] . In Arabidopsis , four RNase Z proteins can process tRNA in vitro [25] : Trz1 and Trz2 (RNase Z L ) localize in the nucleus and mitochondria and may process tRNAs; Trz3 and Trz4 (RNase Z S ) localize in the chloroplasts and cytoplasm, respectively. Loss-of-function of Trz4 leads to embryo lethality, and the function of Trz3, which localizes in the cytoplasm, is largely unknown [25] . The rice genome encodes three RNase Z proteins, including one long form and two short forms (RNase Z S1 and RNase Z S2 ; Supplementary Fig. 7 ). RNase Z S2 localizes in the chloroplast and is essential to chloroplast development [31] . In humans, ELAC2 (RNase Z L ) localizes in the nucleus and mitochondria [32] , [33] . ELAC2 can process the lncRNA MALAT1 and plays a role in the generation of a mammalian herpesvirus microRNA [34] , [35] . ELAC1 (RNase Z S ) occurs in the cytoplasm but has unknown functions [36] , [37] . The enzymatic activity of ELAC2 is over 1,600-fold higher than ELAC1, suggesting that ELAC1 might have new functions other than tRNA processing in the cytoplasm [38] . Our data provide the first direct experimental evidence demonstrating the biochemical roles of a short form of RNase Z (RNase Z S1 ) in mRNA metabolism in the cytoplasm of an eukaryote. Our findings could provide clues to the functions of the RNase Z family not only in plants but also in animals. Plant materials and growth conditions Rice accessions, including AnnongS-1 ( O . sativa ssp. indica , AnS-1, tms5 ), AnnongN ( O . sativa ssp. indica , AnN, WT siblings of AnS-1), Zhonghua11 ( O . sativa ssp. japonica , ZH11, WT), tms5 -ZH11 (the progeny of AnS-1 after two backcrosses to ZH11) and transgenic lines TMS5g-AS (RNase Z S1 transgene in AnS-1 background), TMS5i-ZH (RNase Z S1 RNAi in ZH11 background), Ub L40 1OE ( Ub L40 1 overexpression in ZH11 background), Ub L40 4OE ( Ub L40 4 overexpression in ZH11 background), Ub L40 1i ( Ub L40 1 RNAi in ZH11 background) and Ub L40 4i ( Ub L40 4 RNAi in ZH11 background) were grown in the field under normal conditions at the South China Agricultural University, Guangzhou, or grown in a growth chamber at DATs of 23, 24, 26, 28 and 30 °C ( Supplementary Table 2a ). The photoperiod was 12 h light and 12 h dark, unless specifically indicated. Zhu1S ( O . sativa ssp. indica , tms5 ), 93-11 ( O . sativa ssp. indica , WT), NIL5 and NIL8 (near-isogenic line 5 and 8 of Zhu1S in the 93-11 background), Nipponbare ( O . sativa ssp. japonica ) and transgenic lines TMS5g-ZS (genetic DNA of RNase Z S1 in Zhu1S background) and TMS5i-NB (RNase Z S1 RNAi in Nipponbare background) were planted in the field in Beijing or in Phytotron growth chambers (Koithtron S-153w, Japan) at DAT of 22, 24, 26, 28 and 30 °C with 13.5 h light and 10.5 h dark at the China National Rice Research Institute, Hangzhou ( Supplementary Table 2b ). The rice seedlings were moved to growth chambers or the Phytotron at indicated temperature when panicle length reaches ~1 cm (before the stages of early premeiosis) for ~2 weeks until flowering. All samples from AnS-1 and its controls were harvested between 1500 and 1700 hours in the growth chamber and Zhu1S and its controls were harvested between 0800 and 1100 hours in the Phytotron. Characterization of AnS-1 and Zhu1S phenotypes Rice florets were photographed with an OLYMPUS DP70 digital camera and an OLYMPUS SZX10 dissecting microscope. Mature pollen grains were stained with 1% I 2 –KI solution and observed with an OLYMPUS BX51 or Leica DNRXA microscope. Panicles from various stages of development were fixed with a mixture of 4% paraformaldehyde and 1.5% glutaraldehyde in PBS solution at 4 °C. The samples were then fixed again for 1 h with 1% osmic acid. Fixed anthers were washed three times for 10 min each in PBS solution. After washing, the samples were dehydrated in five successive graded ethanol baths (from 50 to 95%) for 10 min each and then washed in 100% propylene oxide twice for 15 min each. The samples were infiltrated with resin/propylene oxide (1:1 mixture) for 2 h and resin/propylene oxide (3:1 mixture) for 3 h, embedded in pure resin overnight, and then placed in an oven at 60 °C for 48 h. After capsule-embedding, blocks were trimmed on an LKB pyramitome. Trimmed blocks were cut to 2-μm semithin sections on an LKB ultramicrotome with glass knives. The semithin sections were stained with 0.2% toluidine blue O (Chroma-Gesellschaft, Germany) and examined with the Leica DNRXA light microscope or OLYMPUS BX51 microscope. Fine mapping of tms5 and the gene conferring TGMS in Zhu1S The F 2 mapping population was generated from crosses between Xiang125S (derived from AnS-1) and Jingxian 89 ( O . sativa ssp. indica ) and grown in the field during the summer in Guangzhou (DAT>28 °C), Guangdong province in China. The introgressed mapping population (BC 1 F 2 and BC 6 F 2 ) was generated according to the programme shown in Supplementary Fig. 4c and planted in the summer at Changsha (DAT>28 °C), Hunan province in China. Details of the markers used for mapping are listed in Supplementary Table 5 . The candidate genes were sequenced and compared in wild type (AnN and 93-11) and TGMS (AnS-1 and Zhu1S) using the primers shown in Supplementary Table 6 . Vector construction, plant transformation and analysis For functional complementation tests, a 5.3-kb DNA fragment containing 2.3 kb of upstream sequence, the entire TMS5 -coding sequence, and 0.9 kb of downstream sequence, was amplified from AnN genomic DNA using primers TMS5g-AS F/R ( Supplementary Table 6 ), and then digested with BamHI and HindIII and ligated to the binary vector pCAMBIA1300 for gene transformation. A 5.1-kb DNA fragment containing a 2.2-kb upstream sequence, the entire TMS5 gene and a 1.0-kb downstream region from a BAC library (OSJNBb00118O13, Arizona Genomics Institute), was digested with HindIII and ligated to the binary vector pCAMBIA2300 to get the complementary construction, XF2108. For TMS5i-ZH and TMS5i-NB RNAi (construction of XF2114), two DNA fragments (415 and 360 bp, respectively) were cloned from TMS5 cDNA using the primer pairs TMS5i-ZH F/R and TMS5i-NB F/R ( Supplementary Table 6 ), and then inserted into pYLRNAi [39] and pUCC-RNAi [40] . For Ub L40 1 and Ub L40 4 RNAi, two DNA fragments (242 and 322 bp, respectively) were amplified from Ub L40 1 and Ub L40 4 using two pairs of primers, Ub L40 1i F/R and UbL404i F/R ( Supplementary Table 6 ), and inserted into pYLRNAi. For Ub L40 1 and Ub L40 4 overexpression, two DNA fragments (424 bp) from Ub L40 1 and Ub L40 4 were amplified using two pairs of primers, Ub L40 1OE F/R and Ub L40 4OE F/R, and inserted into the pYLox vector [39] driven by the ubiquitin promoter. Transgenic plants were generated via Agrobacterium -mediated transformation [41] , [42] . For each vector, 15 transgenic lines were selected and genotyped. Positive transgenic lines were selected for further analysis by expression level of target genes. Transgenic lines with moderate expression levels were next analysed and average phenotypes were photographed. The relevant PCR primers are listed in Supplementary Table 6 . Subcellular localization The open reading frame of TMS5 was amplified and fused with the N terminus of GFP [43] in the pUC18 vector under the control of the CaMV35S promoter. Protoplasts from leaf sheaths of rice plants were isolated as described previously [44] . Briefly, for protoplast transformation, 10 μl of plasmid carrying TMS5 and GFP fragments, 100 μl of protoplasts and 110 μl of PEG solution (40% PEG4000, 0.3 M mannitol and 0.1 M CaCl 2 ) were mixed gently and incubated for 15 min. After transformation, cells were washed with W5 solution and then resuspended in WI solution (4 mM MES, pH 5.7, 0.5 M mannitol and 20 mM KCl). Cells were incubated ~20–24 h after transformation. GFP signals were observed under the OLYMPUS BX51 fluorescence microscope. Expression analyses Total RNA was isolated from rice roots, stems, leaves, panicles, stamens and pistils at different temperatures using TRIzol (Invitrogen, USA) reagent. DNase I-treated total RNA (2.0 μg) was used for reverse transcription using the M-MLV-RT kit (TAKARA, Japan). RT–PCR and real-time quantitative PCR were performed as previously described [39] , [40] . Briefly, equal amounts of RT products were used to perform PCR. Quantitative PCR analyses were performed three repeats for each sample using the SsoFast EvaGreen Supermix kit (Bio-Rad, USA) with CFX96 Real-Time PCR Detection System (Bio-Rad). The cDNA levels of target genes were normalized to the internal standard genes OsActin1 and OsEF1-α . RNA blotting was performed as previously described [42] . The hybridization signals were visualized using a Typhoon 9000 System (GE, USA). Nuclear and cytoplasmic proteins were purified using Plant Total Soluble Nuclear Protein High-Pure Kit (GENMED, USA). Total protein was extracted from rice panicles grown at different temperatures. Immunoblot analysis was performed using Li’s methods [42] . The complementary sequences corresponding to tRNAs were used as probes labelled with γ- 32 P-ATP using T4 polynucleotide kinase. The hybridization was performed at 42 °C in a hybridizer. The protein extracts were separated by 12% SDS–polyacrylamide gel electrophoresis and transferred to a Pure Nitrocellulose Blotting Membrane (Pall Corporation). The membrane was successively incubated with the anti-RNase Z S1 antiserum (1:1,000 dilution) and secondary antibody goat anti-rabbit IgG HPR (1:10,000 dilution). Actin (Code: M20009; Abmart, China) was selected as the internal standard protein. OsSRT1 (ref. 45 ) and Osβ′-COP [46] were selected as the nuclear and cytoplasmic protein controls. Anti-TMS5, anti-OsSRT1 and anti-Osβ′-COP were generated by immunizing rabbits. The relevant PCR primers are listed in Supplementary Table 6 . Overproduction and purification of RNase Z S1 The RNase Z S1 and RNase Z S1 H81L sequences were amplified (primers see Supplementary Table 6 ) and cloned into plasmid pET23d (Novagen, Germany). After transformation of the E. coli BL21 (DE3) strain with the resulting plasmid constructs in 2 l of LB culture medium at 37 °C, expression of histidine-tagged RNase Z S1 was induced by the addition of 0.1 mM isopropyl-β-d-thiogalactopyranoside and grown at 20 °C overnight. The culture was harvested, pelleted, resuspended in 30 ml of buffer containing lysozyme and stirred for 3 h at 4 °C. The suspension was treated with an ultrasonic disintegrator (SONICS, USA) at 4 °C and then centrifuged at 15,000 g for 30 min to remove cell debris. The supernatant was loaded onto a Ni 2+ -NTA column (Qiagen, Germany). RNase Z S1 was purified using the histidine tag according to the manufacturer’s instructions (Novagen) and immediately dialysed. Protein purity was then verified using SDS–PAGE analysis (12%) and estimated at >95%. Synthesis of tRNA precursors and Ub L40 RNAs in vitro Precursor tRNAs, Ub L40 and CYP86A1 were amplified using specific primers ( Supplementary Table 6 ) and cloned into plasmid pEASY-T3 (Transgene, China). Precursor tRNAs, Ub L40 and CYP86A1 were transcribed in vitro using T7 RNA polymerase and labelled with [α- 32 P]-CTP, according to the manufacturer’s instructions (Promega, USA). The template DNA was removed by the addition of DNase I (Fermentas, USA). The labelled RNAs were purified using phenol and ethanol. RNase Z S1 enzymatic activity assays RNase Z S1 activity was assayed as previously described [24] . Briefly, the labelled precursor tRNAs or Ub L40 RNA were incubated for 0.5, 1, 2 or 4 h at 37 °C with 200 ng purified RNase Z S1 or enzymatic null RNase Z S1 H81L, in which a substitution of histidine by leucine in position 81 in the conserved enzymatic domain of RNase Z proteins causes the loss of enzymatic activity [47] . The RNase Z S1 cleavage products were purified using the RNA probe purification kit (OMEGA, USA). Equal volumes of reactant solutions and 2 × loading buffer (95% formamide, 20 mM EDTA, 0.05% bromophenol blue and 0.05% xylene cyanol) were mixed. Denaturing gel electrophoresis was performed by 8 or 15% PAGE containing 7 M urea and the signals were visualized with the Typhoon 9000 System (GE). RNA ligase-mediated 5′ RACE A 5′ RNA adaptor (5′- CUGACUGCACUCAGAGUACUACAGCCGAC -3′) was ligated to ~2.0 μg of total RNA using T4 RNA ligase 1 (NEB, USA). The ligated mRNAs were then reverse transcribed using oligo(dT) 15 primer with AMV reverse transcriptase (TAKARA). Three rounds of 5′ RACE reactions were performed with two nested primers (outer, CX1544: 5′- GCTGATGGCGATGAATGAACACTG -3′; inner, CX1545: 5′- CGCGGATCCGAACACTGCGTTTGCTGGCTTTGATG -3′) and three gene-specific primers ( Supplementary Table 6 ). The PCR products were gel-purified, cloned (pEASY-T1, Transgen, China) and sequenced. Microarray and RNA-seq analysis RNA samples used for microarray analysis were prepared from young panicles from stages of MMC to meiosis in wild-type (AnN and ZH11) and tms5 (AnS-1 and TMS5i-ZH) plants grown at permissive and restrictive temperatures. RNA purification and Affymetrix microarray hybridization were performed by the Capital Bio Corporation ( http://www.capitalbio.com , Beijing, China). The microarray data were analysed with the Gene Chip Operating software (GCOS 1.4). The different arrays were normalized using DNA-chip analyzer (dChip). The significantly differentially expressed genes between wild-type and tms5 plants were analysed using the Significant Analysis of Microarray software [48] . Single-end 86-nucleotide RNA-seq reads were aligned to the TIGR6.1 genome sequences using TopHat [49] . Uniquely mapped reads were used for subsequent analysis [50] . In situ hybridization analyses Specific regions of RNase Z S1 -, Ub L40 1 - and Ub L40 4 were amplified using corresponding primers ( Supplementary Table 6 ) and then transcribed in vitro as probes using the DIG RNA labeling kit (Roche, Switzerland). Fresh ZH11 young panicles from different developmental stages were fixed immediately, embedded in paraffin (Sigma-Aldrich, USA) and sectioned to 8-μm thickness. Hybridization and immunological detection were performed according to the previously described method [51] . Briefly, sections were over night incubated at 45 °C with coverslips in hybridization buffer (40 μl per slide) containing the probes. Immunological detection of the hybridized probes was performed using a DIG nucleic acid detection kit (Roche) according to the manual. How to cite this article: Zhou, H. et al . RNase Z S1 processes Ub L40 mRNAs and controls thermosensitive genic male sterility in rice. Nat. Commun. 5:4884 doi: 10.1038/ncomms5884 (2014). Accession codes: The microarray and RNA sequencing data have been deposited in the Gene Expression Omnibus (GEO) under the accession codes GSE42367 and GSE42314 , respectively.